Strong-couplingd-wave superconductivity in PuCoGa5probed by point-contact spectroscopy Superconductivity is due to an attractive interaction between electrons that, below a critical temperature, drives them to form Cooper pairs and to condense into a ground state separated by an energy gap from the unpaired states. In the simplest cases, the pairing is mediated by lattice vibrations and the wavefunction of the pairs is isotropic. Less conventional pairing mechanisms can favour more exotic symmetries of the Cooper pairs. Here, we report on point-contact spectroscopy measurements in PuCoGa 5 , a moderate heavy-fermion superconductor with a record high critical temperature T c =18.5 K. The results prove that the wavefunction of the paired electrons has a d -wave symmetry, with four lobes and nodes, and show that the pairing is likely to be mediated by spin fluctuations. Electronic structure calculations, which take into account the full structure of the f -orbital multiplets of Pu, provide a hint of the possible origin of these fluctuations. A century on from the discovery of superconductivity, a complete understanding of some of the mechanisms that lead to its manifestation is still missing. Considerable research efforts are currently devoted to elucidating mechanisms by which pairs of electrons can bind together through the mediation of a boson field different than the one associated with the vibrations of a crystal lattice. PuCoGa 5 , a 5 f -electron heavy-fermion superconductor with a record high critical temperature T c =18.5 K [1] , is one of the many compounds for which the short-range, isotropic attraction provided by simple electron–phonon coupling does not appear as an adequate glue for electron pairing. Magnetic, or virtual valence, fluctuations may have an important role in the stabilization of the superconducting ground state in PuCoGa 5 , but the specific nature of the coupling mechanism remains obscure. PuCoGa 5 is a compound with unique properties. The Sommerfeld coefficient γ , as measured by specific-heat experiments, is between 77 and 95 mJ mol −1 K −1 (refs 1 , 2 ). The effective mass of electrons is about 1/5 of that measured for the isostructural unconventional superconductor CeCoIn 5 [2] , suggesting a smaller degree of electronic correlation. The magnetic properties of PuCoGa 5 and their possible relationship with the superconducting pairing have been debated, mainly because of conflicting results about the magnitude of the magnetic moment carried by the Pu ions. A Curie–Weiss susceptibility in the normal state was initially observed [1] , as expected for fluctuating local Pu 3+ moments. Successive μ SR studies showed no static, normal-state electronic magnetism [3] , [4] , and polarized neutron diffraction experiments showed a small and temperature-independent microscopic magnetization dominated by the orbital moment [5] . The amplitude of the gap Δ (or at least of the gap ratio 2Δ/ k B T c ) has been estimated by different techniques. Using nuclear magnetic resonance (NMR) to measure the Knight shift in the superconducting state of a sample with T c =18.5 K, Curro et al . [6] obtained 2Δ/ k B T c =8 (Δ~6.3 meV). Various band-structure calculations have been reported [7] , [8] , [9] , [10] , [11] , [12] , [13] , [14] , showing that the details of the Fermi surface (FS) and the value of the local magnetic moment in PuCoGa 5 depend on the approximations used to simplify the description of the electron correlations. In the local density/generalized-gradient approximations (LDA/GGA), the FS is quasi-two dimensional (2D) [7] , [8] , [11] , [13] , with at least two nearly cylindrical sheets, one hole-like around the Γ =(0, 0, 0) point of the reciprocal space ( k x , k y , k z ), and one electron-like around M =( π , π , 0). FSs with similar features have been observed in Fe-based superconductors [15] . Indeed, the coupling mechanism that seems to account for the high T c superconductivity in iron pnictides (based on the nesting between hole and electron FS sheets through a vector associated with a peak in the spin susceptibility) had been proposed earlier for PuCoGa 5 [10] . The FS remains qualitatively unchanged with the addition of the Coulomb- U interaction [14] . Several experimental facts [2] , [3] , [6] , [16] , [17] , [18] , [19] suggest that in PuCoGa 5 the electrons in the Cooper pairs have a mutual angular momentum =2, corresponding to a superconducting order parameter (OP) with d -wave symmetry, that is, the gap in the single-particle excitation spectrum has nodal lines intersecting the FS. A direct proof of the gap symmetry is, however, still missing. This is an important point, as the symmetry of the OP is closely related to the pairing mechanism. For instance, while isotropic electron–phonon attraction favors the formation of zero-angular-momentum pairs, with a spherically symmetric OP, d -wave symmetry is most easily realized if the pairing interaction is repulsive at short range and anisotropic at larger distances, as the one provided by effective spin–spin couplings on the border of antiferromagnetism [20] . A magnetic nature of the Cooper pairing mediator in PuCoGa 5 has been discussed by several authors (a recent review can be found in ref. 21 ). Flint et al . [22] considered virtual valence fluctuations of the magnetic Pu configurations, creating Kondo screening channels with different symmetry, and demonstrated that in a lattice of magnetic ions, exchanging spin with conduction electrons in two different channels, a condensate of composite pairs between local moments and electrons is formed. These models must be reconciled with the temperature-independent susceptibility observed in the normal state [5] . A phononic mechanism in the framework of the d -wave Eliashberg theory has been discussed in ref. 19 . Although able to reproduce a number of experimental observations, this model requires an electron–phonon ( e–ph ) coupling constant λ that is much higher than the value experimentally deduced from the time relaxation of photoinduced quasiparticles [23] ( λ =0.20–0.26). To determine the amplitude and the symmetry of the superconducting OP, and thus get some insight into the possible coupling mechanism, we performed point-contact Andreev-reflection spectroscopy (PCARS) measurements in PuCoGa 5 single crystals. PCARS has very often been the key experimental tool to elucidate the unconventional nature of superconductivity in very different materials, from heavy fermions [24] to iron-based superconductors [25] . Based on these PCARS measurements, we prove that the OP of PuCoGa 5 has a d -wave symmetry, consistent with indirect indications from NMR and μ SR measurements. In freshly annealed crystals of 239 PuCoGa 5 with bulk , the analysis of different PCAR spectra gives a gap amplitude at T →0 equal to Δ=5.1±0.3 meV, corresponding to a gap ratio 2Δ/ k B T c =6.4±0.4, that indicates a strong electron–boson coupling. A similar gap ratio is obtained in 242 PuCoGa 5 with Sb impurities and a reduced T c =14.5 K. In both cases, the temperature dependence of the gap is consistent with the predictions of the Eliashberg theory for strong-coupling superconductivity if spin fluctuations provide the mediating bosons. A characteristic boson energy Ω 0 =5.3–8.0 meV (within the range of spin-fluctuation energies determined by NMR) and a coupling constant λ =2.2–3.7 allow reproducing the low-temperature gap values. These results show that PuCoGa 5 is an unconventional, strong-coupling d -wave superconductor and indicate spin fluctuations as the probable boson that mediates the electron pairing. Furthermore, we demonstrate that this picture is not in contradiction with the temperature-independent magnetization. Indeed, electronic structure calculations accounting for the full structure of the 5 f -orbital atomic multiplets and their hybridization with the conduction bands show that the Pu atoms carry non-vanishing average moments as their f shells fluctuate between a singlet and a sextet configuration. These fluctuations are dynamically compensated by fluctuations in the surrounding cloud of conduction electrons such that the compound as a whole remains non-magnetic. 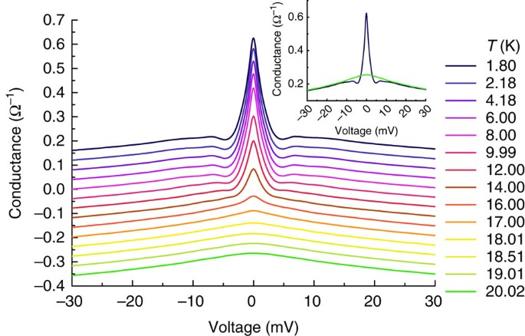Figure 1: Temperature dependence of the experimental conductance curves. Experimental raw conductance curves of a Au/PuCoGa5point contact withRN=6.2 Ω measured at different temperatures. All the curves apart from the top one are vertically shifted for clarity. The inset shows the curve at 1.8 K and the curve at 20.02 K (and thus in the normal state) without any shift. The superposition of the tails is one of the indicators that the contact is in the ballistic regime. Point-contact Andreev-reflection measurements Figure 1 presents the temperature dependence of the raw conductance curves of a point contact whose normal-state resistance is 6.2 Ω. All the curves but the lowest-temperature one are shifted downward for clarity. The top curve is measured at T =1.8 K, which means about T c /10. This ensures that the gap extracted from it is representative of the gap for T →0. The high-energy tails of the conductance curves are temperature independent, as shown in the inset, where the curves measured at T =1.8 K and in the normal state are reported without vertical offset as an example. This demonstrates that the contact is in the perfectly ballistic regime, with no contribution due to Maxwell terms in the contact resistance, that is, there is no diffusion in the contact region and the maximum excess energy with which the electrons are injected into the superconductor is exactly eV . Meeting this condition is essential for energy-resolved spectroscopy to be possible. The absence of heating effects in the contact is also witnessed by the coincidence between the Andreev critical temperature (that is, the temperature at which the Andreev signal disappears and the normal-state conductance is recovered, here between 18.0 K and 18.5 K) and the bulk T c =18.1 K determined from resistivity measurements (as shown in Supplementary Fig. S1 ). Figure 1: Temperature dependence of the experimental conductance curves. Experimental raw conductance curves of a Au/PuCoGa 5 point contact with R N =6.2 Ω measured at different temperatures. All the curves apart from the top one are vertically shifted for clarity. The inset shows the curve at 1.8 K and the curve at 20.02 K (and thus in the normal state) without any shift. The superposition of the tails is one of the indicators that the contact is in the ballistic regime. Full size image It is worth noticing that the normal-state conductance curves in PuCoGa 5 do not show the strong asymmetry observed in various heavy-fermion compounds like, for instance, CeCoIn 5 [26] , UBe 13 [27] and URu 2 Si 2 [28] , [29] (but not, for example, in UPt 3 [30] ). In some cases, this asymmetry was ascribed to magnetic properties of the normal state. In CeCoIn 5 , the asymmetry appears below the temperature where a coherent heavy-fermion liquid develops [26] , and has been explained in terms of a Fano resonance involving localized states near the interface and itinerant heavy electrons in the bulk [31] . The absence of a strong, temperature-dependent asymmetry in PuCoGa 5 may thus confirm that superconductivity in this compound develops out of an incoherent metallic state [32] . In order to compare the experimental curves to the theoretical ones, a normalization is required, that is, a division by the conductance of the same point contact when the superconductor is in the normal state. Owing to the extremely high value of the upper critical field in PuCoGa 5 , this cannot be achieved by applying a magnetic field to suppress superconductivity at low temperature. However, owing to the moderate T c and the negligible temperature dependence of the normal-state conductance (witnessed by the absence of any change in shape of the tails of the conductance curves at | eV |>15 meV), we can safely normalize the conductance curves at any by the normal-state conductance curve measured at (or just above) . The result of this normalization is shown in Fig. 2 (symbols) for two contacts made on different places of freshly broken surfaces of the same sample. The two contacts have the same but different normal-state resistance R N . It is worth noticing that the Andreev signal is very high, while in most heavy-fermion compounds it is suppressed to a few percent of the normal-state conductance [24] , [31] . This effect has been ascribed to extrinsic causes (for example, elastic scattering in the contact region) or intrinsic ones (for example, an energy-dependent quasiparticle lifetime or the existence of unpaired light electrons below T c that do not participate in Andreev reflection [31] ). None of these effects seem to have a role in our point contacts. 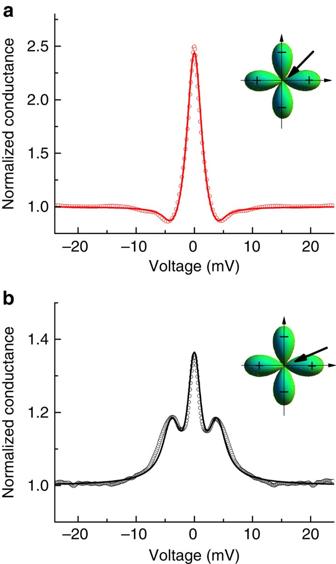Figure 2: Fit of the normalized low-temperature conductance. (a) The conductance curve (measured at 1.8 K) of a Au/PuCoGa5point contact with normal-state resistanceRN=6.2 Ω after normalization (symbols) and the relevant 2D-BTK fit assuming ad-wave gap (line). The parameters of the fitting function are as follows: the gap Δ atT=0 K, the spectral broadening parameterΓ, the measure of the barrier strength at the interfaceZand the angleαbetween the direction of current injection and the direction along which the gap is maximum (that is, it has a lobe). Their values for this curve are Δ=4.85 meV,Γ=0.6 meV,Z=0.84 andα=π/4. The corresponding direction of current injection is shown in the inset. (b) Same as in (a), but for a contact with normal-state resistanceRN=5.5 Ω. The best-fitting parameters are Δ=5.10 meV,Γ=0.8 meV,Z=0.7 andα=π/9.25. The different shape of the two curves in (a) and (b) simply arises from the different direction of the current injected with respect to the lobes of thed-wave symmetry (insets). Figure 2: Fit of the normalized low-temperature conductance. ( a ) The conductance curve (measured at 1.8 K) of a Au/PuCoGa 5 point contact with normal-state resistance R N =6.2 Ω after normalization (symbols) and the relevant 2D-BTK fit assuming a d -wave gap (line). The parameters of the fitting function are as follows: the gap Δ at T =0 K, the spectral broadening parameter Γ , the measure of the barrier strength at the interface Z and the angle α between the direction of current injection and the direction along which the gap is maximum (that is, it has a lobe). Their values for this curve are Δ=4.85 meV, Γ =0.6 meV, Z =0.84 and α = π /4. The corresponding direction of current injection is shown in the inset. ( b ) Same as in ( a ), but for a contact with normal-state resistance R N =5.5 Ω. The best-fitting parameters are Δ=5.10 meV, Γ =0.8 meV, Z =0.7 and α = π /9.25. The different shape of the two curves in ( a ) and ( b ) simply arises from the different direction of the current injected with respect to the lobes of the d -wave symmetry (insets). Full size image The curve in Fig. 2a is similar to the best ones observed in cuprates [33] , [34] , [35] , [36] . Its shape, with a very clear zero-bias conductance peak (ZBCP), whose amplitude is greater than 2, is incompatible with a isotropic OP ( Fig. 3a , top). This is clear in Fig. 3b that reports theoretical curves calculated within the 2D Blonder–Tinkham–Klapwijk (2D-BTK) model for Andreev reflection [37] , [38] , [39] , [40] at a normal metal/isotropic superconductor contact for different values of the dimensionless barrier parameter Z . All the curves present either a plateau or two maxima symmetric about zero bias, and their amplitude is always <2 even in ideal conditions ( T =0, absence of broadening effects). Instead, the experimental curve in Fig. 2a looks very similar to those calculated within the same 2D-BTK model in the case of a nodal OP with a change of sign at the FS. In particular, theoretical curves closely resembling the measured one can be obtained if the OP has a d -wave symmetry (shown in Fig. 3a , bottom), the current is mainly injected along the nodal direction (that is, at an angle α = π /4 with respect to the lobes of the d -wave gap [38] , [39] ) and , as shown in Fig. 3c . In these conditions, the central peak is ascribed to zero-energy Andreev bound states, arising from the constructive interference between electron-like and hole-like quasiparticles that feel OPs with different signs [38] , [39] . 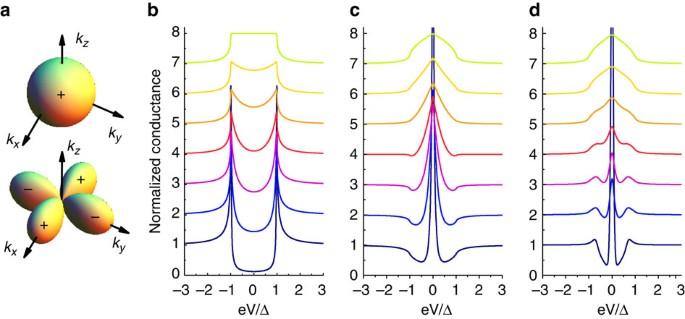Figure 3: Effect of the order parameter symmetry on the Andreev spectra. (a) Plot of the OP in spherical coordinates in the reciprocal space. The cases of ans-wave (top) and of a-wave (bottom) OP are shown. (b) Theoretical normalized conductance curves calculated within the 2D-BTK model atT=0 andγ=0 for a normal metal/s-wave superconductor interface with different values of the dimensionless barrier strengthZ. From top to bottom,Z=0, 0.2, 0.3, 0.5, 0.7, 1.0 and 2.0. (c,d) Normalized conductance curves atT=0 K calculated with the 2D-BTK model for a normal metal/d-wave superconductor interface with the sameZvalues as in (b) and assumingα=π/4 andα=π/8, respectively;αis the angle between the direction of the injected current and thekxaxis. Figure 3: Effect of the order parameter symmetry on the Andreev spectra. ( a ) Plot of the OP in spherical coordinates in the reciprocal space. The cases of an s -wave (top) and of a -wave (bottom) OP are shown. ( b ) Theoretical normalized conductance curves calculated within the 2D-BTK model at T =0 and γ =0 for a normal metal/ s -wave superconductor interface with different values of the dimensionless barrier strength Z . From top to bottom, Z =0, 0.2, 0.3, 0.5, 0.7, 1.0 and 2.0. ( c , d ) Normalized conductance curves at T =0 K calculated with the 2D-BTK model for a normal metal/ d -wave superconductor interface with the same Z values as in ( b ) and assuming α = π /4 and α = π /8, respectively; α is the angle between the direction of the injected current and the k x axis. Full size image The shape of the conductance curve in Fig. 2b is very different, but can be readily explained within the same scenario of d -wave superconductivity if the current is injected along a different direction [38] , [39] . Indeed, this curve looks similar to the theoretical Andreev-reflection spectra calculated within the 2D-BTK model for Z =0.5–0.7 and α = π /8 and shown in Fig. 3d . Fit of the experimental curves Solid lines in Fig. 2a,b are the results of a quantitative fit of the experimental spectra by using the aforementioned 2D-BTK model. The parameters of the model are Δ (here intended as the maximum amplitude of the gap), the barrier strength Z , the angle α and a spectral broadening parameter Γ that must usually be included in the model when fitting experimental curves [40] . Here so that it does not add any ambiguity to the determination of the gap amplitude. The finite experimental temperature (1.8 K) has been taken into account. The best-fitting values of the parameters for the curves of Fig. 2a,b are indicated in the legend. The values of the gap (4.85 meV and 5.10 meV, respectively) are very similar and this is certainly the most important result, but also the barrier and broadening parameters are very similar. The only relevant difference, as expected, is in the value of the angle α , as shown pictorially in the insets of Fig. 2 . 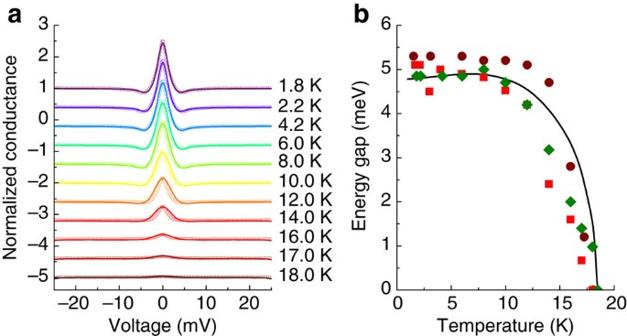Figure 4: Temperature dependence of the gap. (a)Temperature dependence of the normalized conductance curves of a contact withRN=6.2 Ω (symbols) and their fit with the 2D-BTK model (lines). The curves are vertically offset for clarity. (b) Temperature dependence of the gap extracted from the fit of the conductance curves of three different contacts (symbols). The solid line is the Δ(T) function calculated within the Eliashberg theory by assuming a spin-fluctuation-like spectrum peaked at Ω0=6.5 meV and a coupling constantλ=2.37. Figure 4a shows an example of how the normalized conductance curves evolve with increasing temperature. The experimental data (symbols) are compared with the 2D-BTK fit (solid lines). The fit is good at all temperatures; note that both Z and α are independent of temperature and were thus kept constant for all the curves. We also kept Γ nearly constant so that the only parameter that varies significantly with temperature is the gap amplitude Δ. Figure 4: Temperature dependence of the gap. ( a )Temperature dependence of the normalized conductance curves of a contact with R N =6.2 Ω (symbols) and their fit with the 2D-BTK model (lines). The curves are vertically offset for clarity. ( b ) Temperature dependence of the gap extracted from the fit of the conductance curves of three different contacts (symbols). The solid line is the Δ( T ) function calculated within the Eliashberg theory by assuming a spin-fluctuation-like spectrum peaked at Ω 0 =6.5 meV and a coupling constant λ =2.37. Full size image The temperature dependence of the gap as obtained from the fit of three different sets of conductance curves (in three different contacts) is shown in Fig. 4b . It is clear that the gap values are reproducible to a high degree; at low temperature, they range between 4.85 and 5.30 meV. The vertical spread of gap values can be used to evaluate a posteriori the uncertainty on the gap itself; this is obviously much greater than the uncertainty arising from the fit of a single curve, which can be empirically determined as the range of gap values that allow an acceptable (that is, within some confidence limit) fit of the conductance curve, when all the other parameters are varied as well. To be conservative, we can assume the experimental gap at low temperature to be equal to Δ=5.1±0.3 meV, corresponding to a gap ratio 2Δ/ k B T c =6.4±0.4, much larger than the value of 4.28 expected in weak-coupling d -wave superconductors according to the Bardeen-Cooper-Schrieffer (BCS) theory. The spread of gap values is small at low temperature and maximizes at around 14 K. Although the general trend of the gap seems to be compatible with a BCS-like Δ( T ) dependence (but of course, with a non-BCS gap ratio), this uncertainty does not favour discussing it in detail. Analysis of the data within Eliashberg theory The solid line in Fig. 4b , which is in fairly good agreement with the experimental data, represents the theoretical temperature dependence of the gap calculated within the strong-coupling theory for superconductivity (known as the Eliashberg theory [41] , [42] ) by assuming mediating bosons with a spin-fluctuation-like spectrum [43] : where Ω 0 is the energy of the peak and Ω max is a cutoff energy that we chose equal to 4Ω 0 [44] . The shape of the spectrum is shown in the inset of Fig. 5a . In addition to the peak energy Ω 0 , the minimal Eliashberg model contains two other parameters that can be adjusted to reproduce the experimental T c and low-temperature gap: the electron–boson coupling constant λ and the Coulomb pseudopotential μ * (that describes the effects of the Coulomb repulsion and normally ranges between 0 and 0.2 [42] ). The concentration of defects in the material was also taken into account by using a scattering parameter γ d =0.25 meV obtained by fitting the temperature dependence of the local spin susceptibility [6] . 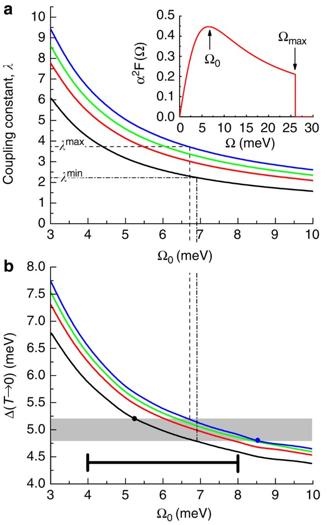Figure 5: Determination of the characteristic boson energy. (a) The electron–boson coupling constantλcalculated as a function of the characteristic boson energy Ω0for selected physically reasonable values of the Coulomb pseudopotential, that is,μ*=0.00 (black),μ*=0.10 (red),μ*=0.15 (green) andμ*=0.20 (blue). The critical temperature is fixed at the experimental valueTc=18.5 K. The concentration of defects in the material was taken into account by using a scattering parameterγd=0.25 meV obtained by fitting the temperature dependence of the local spin susceptibility. The shape of the electron–boson spectral function is shown in the inset. (b) The values of the low-temperature gap Δ(T→0) calculated for all sets of Ω0,λandμ*values corresponding to the curves in (a). The colours of the curves refer to the corresponding value ofμ*, as in (a). The grey region indicates the range of gap values extracted from the point-contact Andreev-reflection measurements. The corresponding range of allowed Ω0is determined by the intersections of the black (minimumμ*) and blue (maximumμ*) curves with the grey region indicated by dots. It turns out that Ω0ranges between 5.3 and 8.5 meV. The maximum and minimum values of the coupling constant compatible with these values areλmin=2.2 andλmax=3.7. The range of spin-fluctuation energies measured by NMR is indicated by the horizontal bar. Figure 5: Determination of the characteristic boson energy. ( a ) The electron–boson coupling constant λ calculated as a function of the characteristic boson energy Ω 0 for selected physically reasonable values of the Coulomb pseudopotential, that is, μ * =0.00 (black), μ * =0.10 (red), μ * =0.15 (green) and μ * =0.20 (blue). The critical temperature is fixed at the experimental value T c =18.5 K. The concentration of defects in the material was taken into account by using a scattering parameter γ d =0.25 meV obtained by fitting the temperature dependence of the local spin susceptibility. The shape of the electron–boson spectral function is shown in the inset. ( b ) The values of the low-temperature gap Δ( T →0) calculated for all sets of Ω 0 , λ and μ * values corresponding to the curves in ( a ). The colours of the curves refer to the corresponding value of μ * , as in ( a ). The grey region indicates the range of gap values extracted from the point-contact Andreev-reflection measurements. The corresponding range of allowed Ω 0 is determined by the intersections of the black (minimum μ * ) and blue (maximum μ * ) curves with the grey region indicated by dots. It turns out that Ω 0 ranges between 5.3 and 8.5 meV. The maximum and minimum values of the coupling constant compatible with these values are λ min =2.2 and λ max =3.7. The range of spin-fluctuation energies measured by NMR is indicated by the horizontal bar. Full size image We first solved the Eliashberg equations in the imaginary-axis representation (explicitly written in the Supplementary Methods ) to determine the pairs of λ and Ω 0 values that, for some given values of μ * between 0 and 0.2, give the experimental T c =18.5 K. In Fig. 5a these pairs are represented by solid lines in the (Ω 0 , λ ) plane. Then, we solved the real-axis Eliashberg equations to calculate the low-temperature gap Δ( T →0) for all sets of Ω 0 , λ and μ * previously determined. The gap values are shown as a function of Ω 0 in Fig. 5b . The range of Ω 0 values that are physically compatible with the PCARS results are finally determined, as shown in Fig. 5b , by intersecting the calculated Δ( T →0) versus Ω 0 curves with the experimental gap range (grey region). The result is . This interval largely overlaps with the range of spin-fluctuation energies (from 4 to 8 meV) determined by NMR measurements [45] ; this clearly indicates that spin fluctuations do possess the right energies to explain the experimental PCARS results. The intersection between the two ranges provides a conservative range for the characteristic boson energy, that is, . The corresponding range of λ values, as shown in Fig. 5 , turns out to be . The line in Fig. 4b was obtained by taking Ω 0 =6.5 meV, μ * =0, and using an electron–boson coupling constant λ =2.37. The slight gap increase at low temperature is a consequence of the strong electron–boson coupling [46] . Further details of the calculations are given in the Supplementary Methods . PCARS measurements on crystals with reduced T c As a test of the reliability and generality of the results discussed so far, we also performed PCARS measurements in 242 PuCoGa 5 crystals featuring a lower bulk , K, due to the presence of Sb impurities (<1%). The point contacts in this case were made by placing a small drop of Ag conductive paste on the side surface of the plate-like crystals. Fig. 6a shows the conductance curves of a Ag/ 242 PuCoGa 5 contact with R N =6.9 Ω measured as a function of temperature. The curves are vertically offset for clarity; as in the cases discussed for the crystals with T c =18.1 K, there is no shift of the tails at increased temperature. The Andreev signal disappears at some temperature between 14.5 K and 14.7 K, that is, . 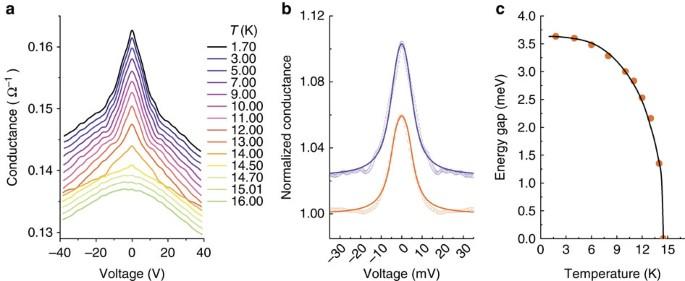Figure 6: PCARS results in crystals with reducedTc. (a) Temperature dependence of the conductance curves of a point contact withRN=6.9 Ω made on a242PuCoGa5crystal with reducedTc=14.5 K. The curves are vertically offset for clarity. (b) Two examples of low-temperature normalized conductance curves in two contacts on the same crystal (symbols). The normal-state resistance and the Andreev critical temperature areRN=6.9 Ω,(top curve) andRN=18.8 Ω,(bottom curve). Lines represent the best fit of the spectra within thed-wave 2D-BTK model. The values of the fitting parameters are: Δ=4.2 meV,Γ=3.7 meV,Z=0.325 andα=π/12 for the top curve, and Δ=3.63 meV,Γ=3.08 meV,Z=0.56 andα=π/11 for the bottom curve. (c) Temperature dependence of the gap extracted from the fit of the conductance curves of the contact withRN=18.8 Ω (symbols). The solid line is the corresponding Δ(T) function calculated within the Eliashberg theory by assuming Ω0=6.5 meV and a coupling constantλ=2.37. Figure 6: PCARS results in crystals with reduced T c . ( a ) Temperature dependence of the conductance curves of a point contact with R N =6.9 Ω made on a 242 PuCoGa 5 crystal with reduced T c =14.5 K. The curves are vertically offset for clarity. ( b ) Two examples of low-temperature normalized conductance curves in two contacts on the same crystal (symbols). The normal-state resistance and the Andreev critical temperature are R N =6.9 Ω, (top curve) and R N =18.8 Ω, (bottom curve). Lines represent the best fit of the spectra within the d -wave 2D-BTK model. The values of the fitting parameters are: Δ=4.2 meV, Γ =3.7 meV, Z =0.325 and α = π /12 for the top curve, and Δ=3.63 meV, Γ =3.08 meV, Z =0.56 and α = π /11 for the bottom curve. ( c ) Temperature dependence of the gap extracted from the fit of the conductance curves of the contact with R N =18.8 Ω (symbols). The solid line is the corresponding Δ( T ) function calculated within the Eliashberg theory by assuming Ω 0 =6.5 meV and a coupling constant λ =2.37. Full size image Figure 6b reports the normalized low-temperature conductance of the same contact (top, symbols) and that of a different contact with R N =18.8 Ω and (bottom, symbols). The shape of these curves, with a zero-bias maximum, confirms that the gap has a d -wave symmetry. It is worth noting that these spectra (as well as all those obtained in crystals with reduced T c ) show a strongly reduced Andreev signal with respect to the ideal case: the excess conductance at zero bias is <10% of the normal-state conductance. A similar effect is commonly observed in heavy-fermion superconductors [24] , [31] and has been reported, in particular, for the isostructural compound CeCoIn 5 [26] , [47] . According to ref. 31 , this reduction might be explained by assuming that a fraction of the injected current tunnels into a non-superconducting band or set of states and does not contribute to Andreev reflection. In our case it seems logical, however, not to ascribe the small signal to intrinsic phenomena but, rather, to the greater amount of disorder and impurities of these samples with respect to the purest crystals (where instead the signal is very high) or to the use of the Ag paste instead of the Au wire as a counterelectrode. In either case, the broadening parameter Γ of the 2D-BTK model can be phenomenologically used to account for extrinsic inelastic scattering. A specific model for diffusive metal/ d -wave superconductor [48] could be used as well, with no major changes in the conclusions. Solid lines in Fig. 6b depict two representative fits of the experimental data within the 2D-BTK model used so far. The fitting parameters are indicated in the legend of the same figure. As expected, the fit requires a large Γ value, although still smaller than the corresponding Δ. Taken all together, the PCARS measurements in these crystals indicate a low-temperature gap Δ=3.9±0.3 meV, corresponding to a gap ratio 2Δ/ k B T c =6.2±0.4. The latter differs only slightly (about 3%) from that determined in the crystals with the highest T c , supporting the robustness of the picture that emerges from our measurements. Figure 6c shows an example of the temperature dependence of the gap extracted from the fit (symbols). The line is calculated within the Eliashberg theory, using the same spectral function and the same values of Ω 0 , λ and μ * as in Fig. 4b . The different T c and the different gap amplitude arise only from the larger value of the quasiparticle scattering rate γ d included in the Eliashberg equations to account for the disorder: while T c =18.5 K was obtained by using γ d =0.25 meV, the reduced T c =14.5 K of this particular contact requires γ d =1.6 meV. This indicates substantial consistency of all the results and generality of the conclusions drawn about the mechanisms of superconductivity in PuCoGa 5 . A scenario where magnetic fluctuations are responsible for the formation of the Cooper pairs in PuCoGa 5 must be reconciled with the observed temperature-independent magnetic susceptibility [5] that points to vanishing local moments at the Pu sites. A plausible explanation is provided by electronic structure calculations combining the LDA with the exact diagonalization (ED) [49] of a single-impurity Anderson model [50] that is composed of a Pu 5 f shell (the impurity) and of those extended states that hybridize with this shell and form the so-called electronic bath. In this approach, the band structure obtained by the relativistic version of the full-potential linearized augmented plane wave method [51] is consistently extended to account for the full structure of the f -orbital atomic multiplets and their hybridization with the conduction bands [52] . Details on this procedure are given in the Supplementary Methods ; the bandstructure and the FS are shown in Supplementary Fig. S2 . The calculated f -orbital density of states (DOS) is shown in Fig. 7 . Below the Fermi energy E F , the DOS exhibits a three-peak structure that is typical for Pu and for a number of its compounds. Our DOS is in reasonably good agreement with the results of the non-crossing approximation reported in ref. 53 and with photoemission experiments performed on single crystals [54] and on thin film samples [55] , as shown in Supplementary Fig. S3 . 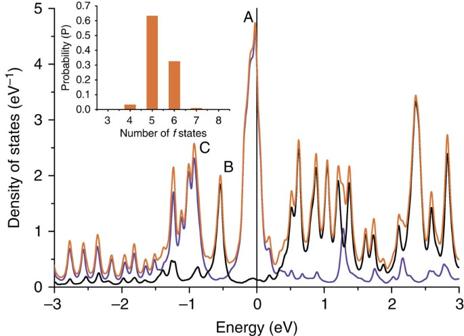Figure 7: Calculated density of states. The 5f-electron DOS at the Pu atom in PuCoGa5(red) and its projections onto the states with the total angular momentumj=5/2 (blue) andj=7/2 (black). Note the three peaks labelled A, B and C that are characteristic for many Pu compounds. The inset shows the valence histogram obtained by the projection of the LDA+ED solution onto the Pu atomic orbitals. Figure 7: Calculated density of states. The 5 f -electron DOS at the Pu atom in PuCoGa 5 (red) and its projections onto the states with the total angular momentum j =5/2 (blue) and j =7/2 (black). Note the three peaks labelled A, B and C that are characteristic for many Pu compounds. The inset shows the valence histogram obtained by the projection of the LDA+ED solution onto the Pu atomic orbitals. Full size image The inset of Fig. 7 shows the valence histogram calculated by projecting the ground state of the Anderson impurity model onto the Pu atomic eigenstates that correspond to an integer 5 f -shell occupation n m . The plotted probabilities P m determine the 5 f -orbital valence The highest obtained probability is P 5 =0.63, followed by P 6 =0.33. In addition, there are small but non-zero probabilities P 4 =0.03 and P 7 =0.01. The Pu 5 f shell has thus an intermediate-valence nature, being a mixture of a magnetic 5 f 5 sextet and a non-magnetic 5 f 6 singlet. Similar electronic structures have been suggested for δ -Pu [56] and several rare-earth-based materials. In the latter case, if the intermediate-valence state involves a non-magnetic atomic configuration, the low- T magnetic susceptibility is temperature independent [57] . The susceptibility of PuCoGa 5 is also found to be temperature independent at low temperatures [5] . The Pu f shell carries a non-vanishing average magnetic moment as it fluctuates between the singlet and the sextet. At the same time, the ground state as a whole is a singlet characterized by all angular momenta equal to zero ( S = L = J =0). The fluctuations of the momenta in the f shell are accompanied by compensating fluctuations in the bath, which can be viewed as a manifestation of the Kondo physics. In analogy to a Kondo singlet state, the magnetic susceptibility is anticipated to behave as , which remains constant for , as observed experimentally [5] . In addition, our band-structure calculations suggest an antiferromagnetic instability due to the presence of a FS sheet with a negative second derivative of the Drude plasma energy, as shown in Supplementary Table S1 . This analysis indicates that the d -wave superconducting coupling in PuCoGa 5 can be mediated by spin fluctuations—even though the microscopic magnetization is temperature-independent—because such fluctuations would involve a time-dependent 5 f local moment dynamically compensated by a moment formed in the surrounding cloud of conduction electrons. Point-contact Andreev-reflection spectroscopy Point-contact spectroscopy is a simple but very powerful tool for the investigation of the superconducting OP that, in past decades, has been successfully applied to many families of superconductors, namely cuprates, borocarbides, heavy fermions and the recently discovered iron-based compounds. The technique consists in measuring the differential conductance of a N–S contact between a normal metal (N) and a superconductor (S) whose radius a is smaller than both the electronic mean free path and the coherence length in S. In these conditions, an electron travels through the contact ballistically, that is, without being diffused, so that if a voltage V is kept at the junction's ends, it enters the superconductor with a maximum excess energy eV . When this energy is smaller than the gap in the superconductor, Δ, the electron cannot propagate in S as an electron-like quasiparticle (ELQ), because it finds no available states. Thus, it forms a Cooper pair and a hole is retro-reflected in N. If the OP is isotropic ( Fig. 3a , top) and there is no potential barrier at the interface, this results in a doubling of the conductance for | V |≤Δ/ e . If | eV |>Δ, the conductance decreases again towards the value it would have if the superconductor were in the normal state. This is shown in the top curve of Fig. 3b , calculated for the case of an ideal barrier-less junction by using the BTK model [37] generalized to the 2D case [39] , [40] . If a potential barrier is present (that is, the dimensionless barrier parameter Z has a finite value), other phenomena take place that can give rise to a normal reflection of the incoming electron, and also to the transmission of hole-like quasiparticles in S. As a result, the conductance presents two maxima at approximately V =±Δ/ e and a zero-bias minimum, as shown in Fig. 3b . If the OP is anisotropic, electrons injected along different directions may experience different pairing amplitudes. Figure 3a (bottom) shows for example an OP with -wave symmetry, , where θ is the azimuthal angle in the k x , k y plane of the reciprocal space and φ is the inclination angle. In cases like this, the shape of the conductance curves does not depend only on the height of the potential barrier at the interface, but also on the direction of (main) current injection with respect to the k -space axes. The curves shown in Fig. 3c,d represent the theoretical conductance curves of a normal metal/ d -wave superconductor calculated by using the 2D-BTK model. In this approach, the FS is supposed to be perfectly cylindrical (with its axis parallel to the k z axis), the dependence of the OP on φ is disregarded, and the direction of current injection is simply defined by the angle α between the normal to the interface n and the k x axis. Note, however, that individual electrons approach the N–S junction from any direction, specified by the angle θ N (0≤ θ N < π /2) between their wavevectors and n [39] . In this paper, in view of the mostly 2D shape of the largest FS sheets (and also for simplicity), we have always used this model. In ref. 40 it is seen that this approximation, with respect to a more refined 3D model, generally gives rise to an overestimation of the parameter Z , which is not relevant in our analysis. If α =0, the normal n is parallel to the k x axis; for any angle of incidence θ N of the incoming electron, ELQ and HLQ transmitted in S with angles + θ S and − θ S with respect to n feel the same OP, in amplitude and sign. However, because of the angular dependence of the gap, the conductance is doubled only at zero bias where it shows a characteristic cusp. If there is no barrier, the same shape is obtained for any value of α : the conductance curve always looks like the top curve in Fig. 3c . If instead a barrier is present, for any α ≠0 some values of θ N exist for which HLQ and ELQ feel OPs of opposite sign [39] . This gives rise to constructive interference between HLQ and ELQ that results in localized zero-energy states (Andreev bound states). These states manifest themselves in the conductance giving rise to a ZBCP. When α = π /4 the current is injected along the nodal direction, all ELQ and HLQ interfere and the ZBCP is maximum. Examples of calculated (normalized) conductance curves assuming α = π /4 and α = π /8 are shown in Fig. 3c,d for increasing values of Z . All the curves in Fig. 3 were calculated at T =0 and in ideal conditions (perfectly ballistic conduction, no broadening effects). When the 2D-BTK model is used to fit experimental data, however, the calculated conductance at T =0 must be convoluted with the Fermi function [40] . Moreover, an additional broadening parameter Γ must be often included in the model to account for the finite lifetime of quasiparticles and other extrinsic broadening effects (like inelastic scattering processes occurring near the N–S interface) [40] . Growth and characterization of the samples The 239 PuCoGa 5 crystals were grown by a flux method and characterized by X-ray diffraction, electrical resistivity, magnetization and specific heat measurements. Magnetic susceptibility and resistivity measurements were performed in commercial Quantum Design platforms (MPMS 7-T SQUID and PPMS-9T). The crystals were submitted to a thermal treatment to anneal the self-radiation damage. Supplementary Fig. S1 shows the temperature dependence of the electrical resistivity measured for one of these crystals immediately after a thermal treatment. All the samples exhibited a critical temperature very close to the optimal value T c =18.5 K. The 242 PuCoGa 5 single crystals were grown from the melt using 242 PuSb instead of metallic 239 Pu as starting material, leading to traces of Sb (<1%) and to a reduced T c =14.5 K. The use of the 242 Pu isotope avoids effects from radiation damage and self heating, especially at low temperature. Magnetization, transport properties and heat capacity confirm their similarity with freshly synthesized single crystals of 239 PuCoGa 5 [5] . Fabrication of point contacts PCARS measurements in 239 PuCoGa 5 were started within 1 day from the thermal treatment. The point contacts were made between a fresh, mirror-like surface of the crystal (just exposed by breaking the sample) and a thin Au wire (about 10 μm in diameter). The uneven broken surface on which the contact is made prevents a fine control of the direction of current injection with respect to the crystallographic axes. However, as shown above, this does not prevent the unambiguous determination of the amplitude and symmetry of the OP. Point contacts in 242 PuCoGa 5 with T c =14.5 K were made on the side surface of the plate-like crystals so as to inject the current mainly along the ab planes. Unlike in the purest samples, here we used a small spot of Ag conducting paste between the Au wire and the sample to act as the N electrode and also to mechanically stabilize the contacts [40] . How to cite this article: Daghero, D. et al . Strong-coupling d-wave superconductivity in PuCoGa5 probed by point contact spectroscopy. Nat. Commun. 3:786 doi: 10.1038/ncomms1785 (2012).